Consistent individual differences in human social learning strategies Social learning has allowed humans to build up extensive cultural repertoires, enabling them to adapt to a wide variety of environmental and social conditions. However, it is unclear which social learning strategies people use, especially in social contexts where their payoffs depend on the behaviour of others. Here we show experimentally that individuals differ in their social learning strategies and that they tend to employ the same learning strategy irrespective of the interaction context. Payoff-based learners focus on their peers’ success, while decision-based learners disregard payoffs and exclusively focus on their peers’ past behaviour. These individual differences may be of considerable importance for cultural evolution. By means of a simple model, we demonstrate that groups harbouring individuals with different learning strategies may be faster in adopting technological innovations and can be more efficient through successful role differentiation. Our study highlights the importance of individual variation for human interactions and sheds new light on the dynamics of cultural evolution. Human success in colonizing nearly all terrestrial habitats of our planet was facilitated by our social nature [1] , [2] . Humans excel in collective action are able to cooperate in social dilemmas and to employ high degrees of group coordination and cooperation to solve adaptive problems. The transmission of information between individuals through social learning was a key factor for the spread of humans across the whole planet [1] . Such cultural transmission has led to the accumulation of huge amounts of adaptive information in very little time. It has been argued that social learning leads to a parallel inheritance system giving rise to a process that is in many ways analogous to genetic evolution [3] , [4] , [5] , [6] . The dynamics and outcome of this process of cultural evolution is to a large extent determined by the rules that govern the transmission of cultural information between individuals, that is, the social learning mechanisms that people use. Several social learning strategies have been described that may each be adaptive under particular circumstances [7] , [8] , [9] , [10] , [11] , [12] . A social learning strategy can specify under which circumstances to pay attention to social information; which individuals to choose as target for collecting information; which type of information to gather from these individuals; and how to use this information as guidance for future behaviour [8] , [13] . Prominent examples of social learning strategies are ‘frequency-based learning’ (for example, to conform to a local majority [3] , [12] , [14] , [15] , [16] ), ‘payoff-based learning’ (to imitate the behaviour of peers who achieved high payoffs in the recent past [3] , [17] , [18] , [19] , [20] ), or ‘prestige-based learning’ (to imitate or follow the advice of high-status individuals such as leaders or teachers [18] , [19] , [20] ). Empirical evidence from the field suggests that these learning strategies do indeed affect the spread of behaviour in human groups [21] , [22] . The results of such investigations are corroborated by evidence from controlled laboratory studies, which indicate that people attend to the frequencies of their peers’ behaviour, as well as to the payoffs associated with it [23] , [24] , [25] , [26] , [27] , [28] , [29] . In addition, there are indications that the extent to which people resort to social information depends on factors like task difficulty, confidence in their own information [30] and environmental variability [31] . Experimental results suggest that individuals differ in the extent to which they rely on social information when making decisions under uncertainty [24] , [28] , and vary in their tendency to conform to behaviour of the majority [26] . As yet, there is no strong evidence that individuals differ with respect to the type of social information that they rely on in making decisions. This is not surprising, since experimental studies of human social information use have predominantly focused on the spread of technological innovations that are mainly relevant in non-social contexts. When attempting to acquire technological know-how, individuals almost exclusively use payoff-based learning (by copying behaviour of successful individuals) when explicitly presented with a choice between multiple social learning strategies [28] . Finding the adequate behaviour in a social setting is quite a different task, which might require different learning strategies. Social ‘know-how’ differs from technological know-how in that the payoffs of the various alternatives do not only depend on the external environment but also on the behaviour of others in the population. When having to choose among alternatives in a non-social setting, the information obtained from others is mainly useful for obtaining a more accurate estimate of the payoffs of these alternatives in a noisy world. In a social setting, these payoffs reflect the behaviour of others. As a consequence, social learning gets a new dimension, namely acquiring information on the distribution of behavioural tendencies in the population. The importance of such frequency information strongly depends on the type of social interaction. Here we study social learning in various social interactions with different signatures. This way we get a more general impression of whether and how social learning differs between technological and social contexts. Moreover, the inclusion of different types of social context allows us to investigate whether individuals are consistent across those contexts. To obtain a better understanding of human social learning in both social and non-social settings, we designed an experiment. Subjects were distributed in groups of eight individuals and experienced four interaction contexts in sequence: a best choice situation (BC; where one of the options yielded a higher payoff on average, irrespective of the behaviour of the other members), a social dilemma (SD; where cooperation is costly to the individual but beneficial for the group), a coordination game (CO; where it is favourable to follow the behaviour of the majority) and an evasion game (EV; where it is favourable to deviate from the behaviour of the majority). Payoffs were noisy, so that it required several trials to find the best option. Before making a decision, all subjects were allowed to request up to six pieces of information about the behaviours and payoffs of their peers, at a small cost (see Methods for details). The information available about each peer included the previous decision, the payoff associated with the previous decision and the total payoff acquired in the current context. We evaluate social learning strategies by tracking the types of information requests that subjects made and by investigating how these requests influenced their behaviour. We demonstrate that individuals differ substantially and consistently with respect to their social learning strategies. Some strongly rely on social information in making their decisions, whereas others tend to learn individually. Those individuals making use of social information differ in the type of information they are interested in: some individuals only focus on the decisions of their group members (thereby neglecting payoff-related information), whereas others consistently request information about both decisions and the payoffs that were associated with them. We repeated our primary experiment in a larger follow-up study to get an impression of the robustness and replicability of our results. Finally, we built a simple model for decision-making in groups to investigate whether individual differences in social learning strategies will affect the direction and outcome of cultural evolution. Dynamics of behaviour and social information use In the course of time, the behaviour in all groups converged to a Nash equilibrium of the game describing the social context ( Fig. 1 , top row, broken lines), indicating that subjects adjusted their behaviour according to the underlying payoff structure (see Methods for details). The availability of social information was associated with a faster adoption of the superior option in the best choice context and the dominant strategy in the social dilemma game ( Supplementary Fig. 1 ). Subjects frequently made use of costly social information ( Fig. 1 ; bottom row; the fraction of decisions preceded by costly request for information was BC: 0.23, SD: 0.25, CO: 0.21 and EV: 0.31). Information requests decreased over time, presumably because there is less need for subjects to adjust their behaviour once their group has approached equilibrium. Individuals usually requested information about only the previous decision ( Fig. 1 , red bars) or the combination of the previous decision and the associated payoff ( Fig. 1 , light blue bars) of their peers. In more than 80% of these cases, requested information entirely consisted of either of those two types; the previous decision of six of their peers or the combination of the previous decision and payoffs of three of their peers (also adding up to the maximally allowed six pieces of information). These types of information requests are consistent with frequency-based learning strategies (such as conformism) and payoff-based learning strategies, respectively. On average, subjects requested social information more often when their own previous decision yielded low payoffs ( Supplementary Fig. 2 ). Also, individuals tended to change their behaviour when information on the behaviour and payoffs of others indicated that alternative behaviour yielded a higher payoff ( Supplementary Fig. 3 ; consistent with payoff-based learning). Reactions to information on the frequencies of peers’ behaviour depended on the interaction context (see Supplementary Fig. 4 ). In the best choice context, the proportion of information requests including requests for payoffs (0.61) was significantly higher than in the social contexts (SD: 0.40, CO: 0.26, EV: 0.33; Tukey contrasts between effect estimates of the factor ‘context’ in a generalized linear model: n =9728 decisions; P <0.001). Subjects requested total payoffs almost exclusively in the last round ( Fig. 1 , dark green, light green, yellow and orange bars), presumably out of curiosity to compare their own performance with that of others. 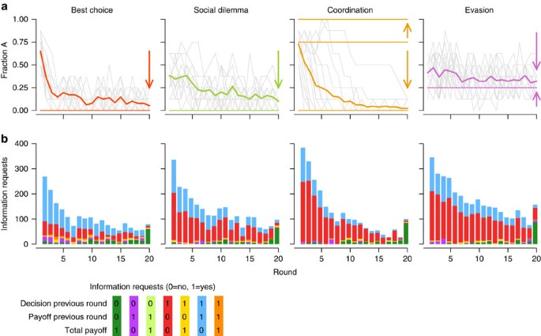Figure 1: Change in behaviour and information requests in the course of time. (a) Change in the relative frequency of cases that optionAwas chosen for each context (sixteen replicate groups in grey, averages in colour). Over time, replicate groups approach a Nash equilibrium of the games (broken lines, arrows; optionByielded a higher payoff thanAin both the best choice and the social dilemma context). (b) Counts of combinations of information types requested in corresponding rounds. Before making their decision, subjects could collect six pieces of costly information about their peer group members. For each peer, available information was his decision in the previous round, his payoff in the previous round and his total payoff obtained in the present context. Requests for payoffs (and associated decisions; light blue bars) prevail in the best choice context and occur regularly in the social contexts; requests only involving recent decisions (red bars) prevail in the social contexts and occur regularly in the best choice context. With the exception of the final round (where subjects often request information on total payoffs) other types of requests are very rare. Figure 1: Change in behaviour and information requests in the course of time. ( a ) Change in the relative frequency of cases that option A was chosen for each context (sixteen replicate groups in grey, averages in colour). Over time, replicate groups approach a Nash equilibrium of the games (broken lines, arrows; option B yielded a higher payoff than A in both the best choice and the social dilemma context). ( b ) Counts of combinations of information types requested in corresponding rounds. Before making their decision, subjects could collect six pieces of costly information about their peer group members. For each peer, available information was his decision in the previous round, his payoff in the previous round and his total payoff obtained in the present context. Requests for payoffs (and associated decisions; light blue bars) prevail in the best choice context and occur regularly in the social contexts; requests only involving recent decisions (red bars) prevail in the social contexts and occur regularly in the best choice context. With the exception of the final round (where subjects often request information on total payoffs) other types of requests are very rare. Full size image Individual variation in social learning strategies Subjects strongly varied in their reliance on social learning. In each context, about 20% of all subjects never requested information ( Fig. 2a ). In contrast, some other individuals based most of their decisions on information about their peers. 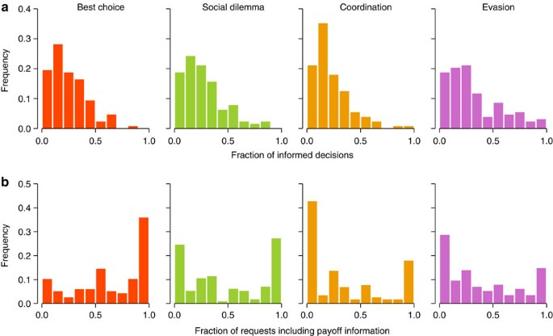Figure 2: Variation among subjects in their reliance on social information and their reliance on payoff information. (a) Distribution of individuals’ reliance on social learning in decision making, measured as the fraction of decisions in which subjects chose to collect peer information. (b) Distribution of individuals’ reliance on payoffs in social learning, measured as the fraction of requests for peer information that included previous payoffs. All distributions are broad and strongly overdispersed when compared with binomial expectations: individuals strongly vary in their reliance on social learning, but even more strongly so with respect to their reliance on payoff information. Figure 2: Variation among subjects in their reliance on social information and their reliance on payoff information. ( a ) Distribution of individuals’ reliance on social learning in decision making, measured as the fraction of decisions in which subjects chose to collect peer information. ( b ) Distribution of individuals’ reliance on payoffs in social learning, measured as the fraction of requests for peer information that included previous payoffs. All distributions are broad and strongly overdispersed when compared with binomial expectations: individuals strongly vary in their reliance on social learning, but even more strongly so with respect to their reliance on payoff information. Full size image The subjects also differed strongly in the degree to which they requested information on payoffs ( Fig. 2b ). While the overall fraction of information requests that included requests for payoffs was intermediate in each context (see above), the underlying individual behaviour was surprisingly extreme. For each context separately, we found that most subjects can be categorized in two largely distinct groups with consistent behaviour: those who rarely include payoff information in their requests and those who do this in the majority of cases ( Fig. 2b ). Consistency of social learning strategies For each of the four contexts, we categorized subjects’ reliance on social learning as low or high when they requested social information in less or more than 25% of the cases, respectively. This cutoff point divided the data in two roughly equal portions for each context (for example, Fig. 2a ). Individuals were significantly more consistent in their reliance on social information (that is, either categorized as ‘high’ or as ‘low’ in all contexts) than expected based on independence between contexts ( Fig. 3a ). Subjects showed a similar consistency with regard to the type of social information they relied on; many of them either strongly relied on payoff-information across all contexts ( Fig. 3b , red bar) or hardly relied on payoff-information at all ( Fig. 3b , blue bar; an individual’s reliance on payoffs was categorized as ‘low’ or ‘high’, depending on whether her information requests included payoffs in less or more than 50% of the cases). The abundance of these consistent individuals was much higher than expected based on independence between contexts (subjects with consistent high and low reliance on payoffs occurring 6.13 and 2.77 times more than expected on the basis of independence, respectively; χ 2 =9.811, n =128, d.f.=1, P =0.002, and χ 2 =7.093, n =128, d.f.=1, P =0.008). Another large fraction of subjects employed a specific flexible social learning strategy, with high reliance on payoffs in the (non-social) best choice context and low reliance on payoffs in the other (social) contexts—this is the social learning behaviour that one might intuitively expect (see introduction). However, these ‘sensible switchers’ are not more abundant than expected based on independence between contexts ( χ 2 =0.319, n =128, d.f.=1, P =0.572). We did not observe significant differences between types of social learning strategies and performance in the experiment, as reflected in total earnings (Tukey contrasts on a linear model: n =128, P >0.121 for comparisons between the three types of social learners highlighted in Fig. 3b ). 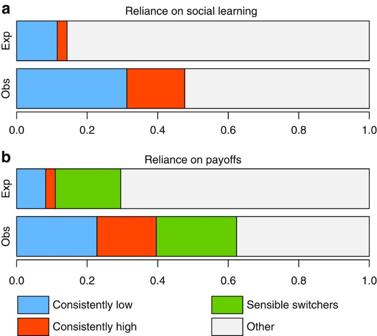Figure 3: Individual consistency across contexts in reliance on social information and reliance on payoff information. (a) For each of the four contexts, we categorized subjects according to their reliance on social learning as low (<0.25) or high (>0.25), resulting in a quadruple of low-high values. The observed fraction of individuals with consistent (‘always high’ or ‘always low’) reliance on social learning is significantly larger than expected on the basis of independence across contexts (χ2=24.725, d.f.=1,n=128,P<0.001). (b) Similarly, subjects were categorized for each context according to their reliance on payoffs in social learning (low <0.5, and high ≥0.5). The observed fraction of individuals with consistent reliance on payoffs is significantly larger than expected (χ2=20.436, d.f.=1,n=128,P<0.001). The figure also shows the observed and expected frequency of ‘sensible switchers’ (individuals categorized as high in the best choice context and as low in the three social contexts). In bothaandb, the ‘other’ category contains the remaining combinations of low-high values, none of which had a frequency >0.1. Figure 3: Individual consistency across contexts in reliance on social information and reliance on payoff information. ( a ) For each of the four contexts, we categorized subjects according to their reliance on social learning as low (<0.25) or high (>0.25), resulting in a quadruple of low-high values. The observed fraction of individuals with consistent (‘always high’ or ‘always low’) reliance on social learning is significantly larger than expected on the basis of independence across contexts ( χ 2 =24.725, d.f.=1, n =128, P <0.001). ( b ) Similarly, subjects were categorized for each context according to their reliance on payoffs in social learning (low <0.5, and high ≥0.5). The observed fraction of individuals with consistent reliance on payoffs is significantly larger than expected ( χ 2 =20.436, d.f.=1, n =128, P <0.001). The figure also shows the observed and expected frequency of ‘sensible switchers’ (individuals categorized as high in the best choice context and as low in the three social contexts). In both a and b , the ‘other’ category contains the remaining combinations of low-high values, none of which had a frequency >0.1. Full size image Robustness and replicability To check for the robustness and replicability of the results obtained, we conducted a follow-up experiment that shared the same general setup with the primary experiment but differed in various aspects (group size was five instead of eight, individuals were allowed to view only four pieces of information per round, the payoff matrices were slightly different, the stochastic component in the payoffs was increased; see Methods for details). In general, our follow-up experiment confirmed all main results of the primary experiment. As in the primary experiment, groups approached the Nash equilibria of the one-shot version of the games in all four contexts ( Supplementary Fig. 5 ). Again, most requests were for either a combination of previous decision and associated payoffs or for previous decisions only. In all four contexts, subjects tended to request information more often in the follow-up experiment (ANOVAs; BC: P =0.035; SD: P <0.001; CO: P =0.071; EV: P <0.001, n =328 for each test). Since the stochasticity in payoffs was higher in the follow-up experiment, this finding is in line with results reported in the literature (for example refs 30 , 31 ). As in the primary experiment, subjects varied strongly in the extent to which they based their decisions on social information ( Supplementary Fig. 6 ). When requesting information, individuals again differed substantially in the type of information they were interested in; some always included payoff information in their requests, whereas others ignored payoff information altogether. These differences among individuals were even more pronounced in the follow-up experiment than in the primary experiment. As in our primary experiment, we find ( Supplementary Fig. 7 ) that the fraction of individuals that was consistent in their social information use is significantly larger than expected on the basis of independence ( χ 2 =29.551, n =200, d.f.=1, P <0.001). This is also the case for individuals’ consistency in reliance on payoffs ( χ 2 =13.673, n =200, d.f.=1, P <0.001). In other words, as in our primary experiment, many individuals were consistent in either strongly or weakly relying on social information, and many individuals were consistent in the type of social information they requested. Implications of individual variation for cultural evolution Our experimental results indicate that there are strong and consistent individual differences in social learning strategies. But does this individual variation matter? To address this question, we developed a simple model of cultural evolution in which individuals interact in small groups and are allowed to update their behaviour by either payoff-based learning (by imitating peers who achieved high payoffs) or frequency-based learning (by imitating the majority). We imposed two conditions: a homogeneous population, in which all individuals updated their strategy by payoff-based learning or frequency-based learning with a 50–50 probability, and a heterogeneous population, in which half of the individuals in a group always updated based on payoffs, and the other half always updated based on frequencies. In our simulations, we documented the fixation probability of behaviour A or B after the introduction of a single B mutant in a population of A players. 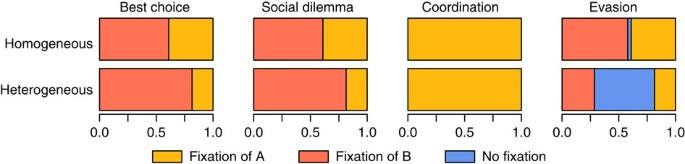Figure 4: Effect of diversity in social learning strategies on the outcome of cultural evolution. For each of the four contexts, we simulated groups of eight individuals that were allowed to update their behaviour using payoff-based or frequency-based learning (tendencies to copy either successful or popular behaviour, respectively). Pairs of bars present the state of the groups after 160 iterations (corresponding to the 20 rounds of our experiments) when initialized with oneBplayer in a group ofAplayers (105replicates each). The top row of bars shows the outcome in homogeneous groups, where each individual uses either form of learning with equal probability. The bottom row of bars shows the outcome in case of heterogeneous groups, where four individuals always use payoff-based learning, while the four others always use frequency-based learning. Individual variation can cause groups to adopt superior technologies (optionB) more readily in a best choice context, but cooperation (optionA) tends to be less stable in a social dilemma. Moreover, in heterogeneous groups,AandBcoexist more stably in an evasion game. Figure 4 shows the outcome of simulations after an average of 20 updates per individual (in correspondence to the number of rounds in the experiments). In three out of four contexts, the existence of individual variation in social learning strategies considerably affects the outcome of cultural evolution. In the coordination game, payoff-based and frequency-based learning both disfavour the spread of rare behaviours, so B will be rapidly lost both in homogeneous and heterogeneous populations. In the best choice context, a newly introduced superior technology ( B ) is more likely to reach fixation in heterogeneous populations; payoff-based learners readily adopt B , and the increase in frequency of B reduces the risk that the superior technology disappears due to frequency-based learning or stochastic processes (for example, copying errors). The same logic applies to the social dilemma: a newly introduced ‘cheater’ mutant will obtain higher payoffs, and payoff-based learners in a heterogeneous population will readily switch to defection; once cooperators are no longer in the majority, frequency-based learners start defecting and cooperation is lost. In the evasion game, variation in social learning strategies enhances the stability of the coexistence of A and B . When assuming the same noise on payoffs as in the primary experiment, the mean time until fixation of either behaviour is increased by 50% in groups that are heterogeneous with respect to social learning strategies, compared with homogenous groups. When payoffs are less noisy the strength of this effect increases, further stabilizing the coexistence of different behaviours. The emerging role differentiation can thus increase average payoffs in a group. Interestingly, in heterogeneous populations, social learning strategies become correlated with behaviour in this game (playing A or B ; see Supplementary Figure 8 , and Supplementary Note 1 for model details and additional model analyses). Figure 4: Effect of diversity in social learning strategies on the outcome of cultural evolution. For each of the four contexts, we simulated groups of eight individuals that were allowed to update their behaviour using payoff-based or frequency-based learning (tendencies to copy either successful or popular behaviour, respectively). Pairs of bars present the state of the groups after 160 iterations (corresponding to the 20 rounds of our experiments) when initialized with one B player in a group of A players (10 5 replicates each). The top row of bars shows the outcome in homogeneous groups, where each individual uses either form of learning with equal probability. The bottom row of bars shows the outcome in case of heterogeneous groups, where four individuals always use payoff-based learning, while the four others always use frequency-based learning. Individual variation can cause groups to adopt superior technologies (option B ) more readily in a best choice context, but cooperation (option A ) tends to be less stable in a social dilemma. Moreover, in heterogeneous groups, A and B coexist more stably in an evasion game. Full size image Cross-cultural experiments have established that human social behaviour strongly varies between cultures [32] , [33] . This suggests that considering the behaviour of typical (‘WEIRD’ [34] ) participants in decision making experiments is likely to lead to an underestimation of the variation present in the human population. Our experiment shows that even within such a relatively homogeneous sample of subjects there is strong and consistent variation in the way people behave. The pronounced individual differences in social learning strategies we report emphasize that the average behaviour in a group or population is far from representative for the behaviour of its constituent individuals. Furthermore, our simulation model suggests that individual variation can affect the dynamics and outcome of social interactions. Although individual differences have been at the heart of personality research in psychology (for example, ref. 35 ), they are often disregarded in many other areas of the social sciences. Our results strongly suggest that individual differences need to be taken seriously, both in theoretical models and in the analysis of empirical data. More specifically, we advocate that models of cultural evolution take individual differences in social learning strategies into account. In the best choice context, the availability of social information was associated with an increase in the adoption of the optimal behaviour. This is in line with earlier findings in the experimental and theoretical literature that social learning can increase an individual’s performance in non-social contexts [3] , [9] , [26] . The way in which social information was used in this context substantially differed between individuals, which is in agreement with earlier experimental evidence [24] , [26] . Our experimental results indicate that individual variation in social learning strategies is even more pronounced in social contexts, where payoffs depend on the behaviour of others. Of course, the results of highly stylized experimental study like ours should not be over-interpreted. Decision-making experiments in a lab setting allow for a high degree of control, but inevitably abstract from potentially important aspects of reality. Although our experimental design imposed relatively few restrictions on how individuals could track their social environment, our study does not account for a variety of factors that play a role in real-life cultural transmission. For instance, it was impossible for subjects to bias their attention towards older, more experienced or more dominant peers [21] , [36] , [37] , and active teaching [38] was excluded by design. Also, subjects were unable to control the accessibility of information about their own behaviour and payoffs [27] . Moreover, subjects in our experiment were informed about the general structure of the interaction contexts in which they were interacting. In reality, this structure is typically unclear and people have to base their decisions on their best guess of how their behaviours and the behaviour of others affect their payoffs. More specific to our design including different contexts, subjects in a session always encountered the simplest (non-social) best choice situation first and subsequently interacted in the other (social) contexts in random order. Some of these concerns can be addressed by additional experiments. Still, whereas laboratory experiments can unravel interesting features of human behaviour, they only present a first step: these aspects should subsequently be scrutinized under more realistic conditions. Assuming that the individual variation found in our study is ‘real’, why should individuals differ in their learning strategies and why should they be consistent in their use of social information across different contexts? Possible explanations can be found in the literature on ‘animal personalities’. In recent years, evidence has accumulated that consistent individual differences in behaviour (‘behavioural syndromes’ or ‘personalities’) are not only prevalent in humans, but also exist throughout the animal kingdom [39] , [40] . In the past, it has often been assumed that selection on behaviour should result in a single, optimally adapted phenotype. By studying animal personalities, it has become apparent that a variety of mechanisms (reviewed in ref. 41 ) can lead to the evolutionary emergence of consistent individual variation in behaviour. More specific models based on this theoretical framework predict the coexistence of alternative life history strategies [42] , [43] ; the coexistence of individuals differing strongly in responsiveness and social sensitivity [44] , [45] ; and the coexistence of different communication strategies [46] . These results may serve as a useful starting point for understanding the consistent individual differences in social learning strategies observed in this study. Cognitive constraints and incomplete information on the learning context will often prevent the evolution of learning strategies that are optimal in every possible circumstance. Instead, evolution may result in the coexistence of locally suboptimal but cognitively ‘cheap’ strategies using rules-of-thumb (for example, ref. 47 ) such as payoff-based learning or frequency-based learning. Other mechanisms facilitating the coexistence of behavioural strategies may apply to social learning as well. For example, the benefits of information are often negatively frequency dependent: the value of information decreases when more individuals also have this information. This immediately explains why individuals relying heavily on information coexist with others that are seemingly not interested in gathering information at all [44] . Last, but not least, the coexistence of learning strategies could be explained by ‘synergy’ between different forms of learning. As suggested by our simulation model, group heterogeneity with respect to learning strategies may under some circumstances lead to more efficient outcomes. Such synergetic effects might again induce negative frequency-dependent selection and result in the coexistence of alternative learning strategies. Even if different learning strategies do coexist, one might expect that individuals are flexible and employ different strategies in different contexts. Again, the literature on animal personalities has revealed various mechanisms explaining a more rigid behaviour, corresponding to the consistent use of the same type of behaviour in different contexts. Behavioural consistency can be favoured when strategic conventions are establishing [48] or when behaviour serves as a signal to others. For example, already a small fraction of ‘socially responsive’ individuals in a population may exert a strong selection pressure in favour of consistency [45] . Consistency can also be supported by all kinds of positive feedbacks: individuals can increase their performance with the consistent use of a certain social learning strategy, due to an increased efficiency in the collection, interpretation and application of the kind of information as they get more experienced in using this strategy. Rather than explaining individual variation from an evolutionary perspective, scholars of human personality have focused on characterizing the structure of individual differences. This has resulted in a number of models that aim to describe human personality along a few dimensions (the ‘Five Factor Model’ [49] being best-known example). It is not unlikely that the observed variation in social learning strategies is associated with these dimensions or factors, and this possibility presents an interesting objective for further research. For instance, one might predict that reliance on social information is associated with openness or with an orientation towards collectivism (as opposed to individualism [50] ); in fact, this latter association has recently been reported by Toelch and colleagues [51] . Similarly, one might expect that individuals who focus on payoff-information are inclined to behave more competitively (rather than cooperatively) in social interactions. To our knowledge, there is no empirical evidence showing how social learning strategies themselves transmit between individuals. As a result, a discussion about the origin of the individual differences we report is highly speculative. In humans as well as in other animals, personality traits often have a high heritability [52] , [53] , and the same might apply to social learning strategies. The expression of social learning strategies may be strongly affected by the environmental conditions during individual development. When parents and their offspring grow up in different environments, their orientations towards individualism/collectivism can differ substantially [54] , and the same could be the case for social learning strategies. Such plasticity is possible even in case of a strong genetic basis, provided that the expressed learning strategy reflects a heritable norm of reaction (where the genotype determines how a trait is expressed in response to the environment [41] , [55] ). In humans, parents often have a strong influence on the development of social tendencies in their children [56] , and this might also apply to social learning. In other words, social learning strategies might themselves be acquired through social learning [57] . If individuals do indeed differ systematically and consistently in their social learning strategies (as our study suggests), carefully designed cross-generational studies could provide valuable insights into the origins of these differences. Another interesting future direction would be to address whether the presence of individual differences in social learning strategies affects the behavioural dynamics of a group (as predicted by our simulation model). One could experimentally test this by creating groups of individuals assorted according to their social learning strategies, and comparing these homogeneous groups to unassorted (heterogeneous) groups. Another interesting question that could be tested in such a setup is whether the behavioural dynamics are different between groups that are homogeneous for different social learning strategies (such as payoff-based learning and frequency-based learning). For example, one might expect that a group of payoff-based learners more readily adopts new superior technologies, whereas groups of frequency-based learners are faster in reaching equilibrium in a coordination context. In eight independent sessions of our first experiment (the ‘primary experiment’), we confronted sixteen subjects ( n =128) with four settings (‘contexts’). In each context, the subjects had to make choices between two options A or B , but the contexts differed in the way payoffs depended on the subject’s own decision and the decisions of others. We based our design on the experimental paradigm of McElreath et al. [24] , and we extended this setup to include interactions in the three strategically different classes of games with pure strategies [16] , each of which has been extensively researched in the literature on the evolution of cooperation [58] . Each subject sequentially encountered a best choice (BC) situation where one option ( B ) yields on average a higher payoff; a social dilemma (SD) where one option ( A ) increases the payoffs of all group members but in each situation yields a lower payoff than the other option ( B ) for each individual employing it; a coordination game (CO), where the payoff of each option ( A or B ) increases with the number of subjects employing this option; and an evasion game (EV), where the payoff of either option ( A or B ) decreases with the number of subjects choosing this option. The best choice context corresponds to a non-social (technological) decision situation, while the other three contexts represent different types of social settings. Decision making was formulated as planting crops on the land of an imaginary farm. In each of the twenty rounds of each interaction context, subjects could decide which of two crops they would plant on their farm (we used actual crop names, but for simplicity we will refer to the options as A and B ). Payoffs were noisy, so that it would require several trials to find out which option was better (see below for details). In each round, subjects had to decide simultaneously and anonymously for one of the two options. Before making their decisions, subjects could pay a small cost to collect information about their peers. The information available about each peer included the previous decision, previous payoff and the total payoff acquired in the current context. If a subject chose to collect information, she could freely request up to six pieces of information. For example, a subject might request all three types of information of two (out of seven) of her peers, or she might request only the previous decision of six of her peers. At the end of each round, subjects were informed about their own payoff in that round. As a benchmark, we ran four control sessions with sixteen subjects each ( n =64), in which subjects could not collect social information from their peers before making their decision. Otherwise, the setup of these sessions was identical to the setup of our primary experiment. In Supplementary Fig. 1 , we report on the findings of the control sessions. To check for the replicability and robustness of the results obtained, we also conducted a second experiment (the ‘follow-up experiment’), consisting of 10 sessions with 20 subjects each ( n =200). The basic setup of this follow-up experiment was the same as the primary experiment reported in the main text: we confronted participants with four interaction contexts in sequence, each consisting of a block of 20 rounds. In each round, subjects made a decision between two options, and, before making their decision, subjects could collect social information about their peers. However, there were a few differences with the primary experiment. First, subjects interacted in groups of five instead of eight; second, because the group size was not the same, the payoff matrices were changed (see below); third, the stochastic component of the payoffs was larger (also, see below); fourth, the maximum number of pieces of information subjects could collect in a round was limited to four, instead of six; finally, subjects could no longer request information about the total payoffs of their group members, but only about their previous decisions and previous payoffs. Earnings and experimental details In total, we ran 22 independent experimental sessions with n =396 subjects. Subjects were recruited using the database of the Sociological Laboratory of the University of Groningen. Participation was by informed consent, and the experimental setup was approved by the Sociological Laboratory of the University of Groningen. Subjects (132 male, 264 female; aged 18 to 31, mean age 22) were mostly undergraduate students from the social sciences, economics and biology. Experimental sessions lasted around 90 min, in which subjects earned [euro]29.60 on average according to their performance, excluding a show-up fee of [euro]5. Instructions were handed out in the reception room of the laboratory and read out loud by one of the experimenters. Each participant received a randomly chosen number corresponding to a desk in the laboratory. Before the experiment itself started, subjects played a test trial of five rounds, making them familiar with the decision-making environment. After that, four blocks of 20 rounds were started, each presenting a different context of social interaction. At the beginning of each block of rounds, specific instructions for the upcoming interaction context were given on the computer screen and participants had to fill out a brief quiz to check their understanding (see Supplementary Note 2 for instructions on paper, and on-screen instructions, including screenshots). Subjects were randomly grouped, labelled with a number 1–8, and each received 3,000 points to play with (1,000 points=1 euro). During the block of rounds, subjects could make substantial profits, but subjects could also lose their initial endowment in case of negative outcomes. After a block of twenty rounds ended, new groups were formed, and subjects were informed about the payoff structure of the new context (again followed by a short quiz). Sessions finished with a questionnaire including items about personal demographic background. Participants were paid individually in the reception room. The experiment was conducted using Z-Tree [59] ; code is available upon request. Subjects were always confronted with the ‘best choice’ context first. Starting with this most simple interaction context facilitated the subjects’ understanding of the context they were in and how their decisions affected their payoffs. The three other interaction contexts–in which payoffs depended on the decisions of others–were played in randomized order. These other contexts correspond to the three different classes of games: a social dilemma, a coordination game and an evasion game. Interaction contexts Each of the interaction contexts was characterized by a payoff matrix . This means that the deterministic component of the payoff of a subject choosing A and B was given by p·a +(1− p )· b and p·c +(1− p )· d , respectively, where p denotes the relative frequency with which A is chosen in the group. The payoff matrices were chosen such that at p =0.5, the payoff difference between A and B was equal in each of the interaction contexts. In the best choice context (BC), a subjects’ payoff did not depend on the decisions of the other subjects in their group ( a = b and c = d ); the payoff matrix was given by . Irrespective of the behaviour of the other players, option B yielded higher payoffs on average. In game theoretical terms, B dominates A and therefore p *=0 is the Nash equilibrium of the one-shot version of the ‘game’. In the social dilemma (SD), cooperation ( A ) is dominated by defection ( B ): a < c and b < d ; the payoff matrix was given by . Therefore, like in the best choice context, p *=0 was the Nash equilibrium of the one-shot version of the game. However, all subjects obtain a higher payoff when they all cooperated ( p =1), compared with this equilibrium ( a > d ). This shows that, in this context, collective interests and individual interests are opposed to each other, like in the famous (two-player) Prisoner’s Dilemma game. In the coordination game (CO), the payoff of choosing one of the two options increased with the number of others also choosing it ( a > c and b < d ). The payoff matrix was given by . In this case, both p *=0 and p *=1 are Nash equilibria. However, the Nash equilibrium at p *=0 is Pareto superior; the payoff to all players was higher compared with the equilibrium at p *=1. There was an (dynamically unstable) equilibrium located at p *=( d − b )/( a − b − c + d ). In this equilibrium (in our case, when two subjects chose A and six subjects chose B ), the expected payoffs of choosing A and choosing B were equal, but any deviation from this equilibrium leads towards either of the Nash equilibria. Typical examples of coordination games are the Stag-hunt game and the Battle of the Sexes [60] . In the evasion game (EV), the payoff of choosing one of the two options decreased with the number of others also choosing it ( a < c and b > d ). The payoff matrix was given by . In this case, there was a Nash equilibrium given by equation p *=( d − b )/( a − b − c + d ), where, in our case, two subjects choose A and six subjects choose B . Typical examples of evasion games are the Hawk-Dove game and the Snowdrift game [61] . In the follow-up experiment, the interaction contexts were characterised by the following payoff matrices: best choice: , social dilemma: , coordination game , evasion game . As in the primary experiment, we chose the parameters such that, at p =0.5, the payoff differences between A and B are equal (that is, 200) in each of the interaction contexts. In the coordination game, the unstable equilibrium was situated where three players choose A and two players choose B. The Nash equilibrium of the one-shot version of the evasion game was situated where two players chose A and three chose B. All other equilibria were the same as in the primary experiment. Payoffs were noisy, reflecting the fact that the outcome of behaviour is often influenced by exogenous factors. This noise made it harder for the subjects to find out individually which choice was optimal, and, as a consequence, made social information more valuable. Noise was implemented by adding a stochastic term to the deterministic component of the payoffs of each subject separately. This stochastic component was a number drawn from a normal distribution with mean 0 and s.d. σ . In the primary experiment, we set σ =175, so that at p =0.5, choosing the option with the lower expected payoff nevertheless leads to higher payoffs in 16% of the cases. In the follow-up experiment, the stochastic component on the subjects’ payoffs was relatively larger than in our primary experiment ( σ =200). This implies that at p =0.5, choosing the inferior option nevertheless leads to higher payoffs in 24% of the cases. Simulation details Details of the model of cultural evolution can be found in Supplementary Note 1 . How to cite this article : Molleman, L. et al. Consistent individual differences in human social learning strategies. Nat. Commun. 5:3570 doi: 10.1038/ncomms4570 (2014).